Optofluidic laser for dual-mode sensitive biomolecular detection with a large dynamic range Enzyme-linked immunosorbent assay (ELISA) is a powerful method for biomolecular analysis. The traditional ELISA employing light intensity as the sensing signal often encounters large background arising from non-specific bindings, material autofluorescence and leakage of excitation light, which deteriorates its detection limit and dynamic range. Here we develop the optofluidic laser-based ELISA, where ELISA occurs inside a laser cavity. The laser onset time is used as the sensing signal, which is inversely proportional to the enzyme concentration and hence the analyte concentration inside the cavity. We first elucidate the principle of the optofluidic laser-based ELISA, and then characterize the optofluidic laser performance. Finally, we present the dual-mode detection of interleukin-6 using commercial ELISA kits, where the sensing signals are simultaneously obtained by the traditional and the optofluidic laser-based ELISA, showing a detection limit of 1 fg ml −1 (38 aM) and a dynamic range of 6 orders of magnitude. Enzyme-linked immunosorbent assay (ELISA) is one of the most popular and powerful analytical methods for biomolecular analysis. In one of the common ELISA formats, sandwich ELISA, capture antibodies are first immobilized on a glass or plastic surface. The target analytes are added and captured to the solid surface. Then the secondary antibodies labelled with enzymes are added and bind to the target analytes, followed by addition of substrates. The fluorescence generated from the product of the enzyme-substrate reaction is detected and its intensity is used to quantify the enzymes and hence the analytes attached to the solid surface. Sensitive detection of the target analytes with a large dynamic range is highly desirable in many applications such as early diagnosis and monitoring of diseases, where the analyte concentration is extremely low and may vary orders of magnitude depending on the physiological condition of a patient [1] , [2] , [3] . However, the traditional light intensity-based ELISA detection suffers from various types of noises, such as those caused by non-specific bindings, autofluorescence of materials and leakage of excitation light, and so on, all of which significantly deteriorate the ELISA performance in detecting ultra-low concentrations of analytes and limit its dynamic range. Recently, ELISA using various microfluidic and photonic structures such as plasmonics and photonic crystals has been explored in an attempt to enhance the fluorescence intensity [4] , [5] , [6] . Detection limits on the order of femto-molars were demonstrated. Digital ELISA was also developed to further advance the sensing performance beyond that of the traditional ELISA. It used hundreds of thousands of beads, each having on average a fraction of an analyte on its surface, to detect the analyte down to sub-atto-molar concentrations [7] . Furthermore, combination of digital and traditional ELISA enabled a dynamic range of 6 orders of magnitude [3] . However, in order to achieve the superior sensitivity this method requires low non-specific bindings to ensure the number of non-specifically bound enzymes on each bead far lower than one. The sensing capability degrades over 1,000-fold in the presence of higher non-specific bindings from serum [7] . Moreover, careful adjustment of the bead-to-analyte ratio and complicated statistical analysis are needed, making the experiment and data interpretation less straightforward. Here we develop the optofluidic laser-based ELISA. The optofluidic laser is an emerging technology that integrates microfluidics, optical microcavity and laser gain medium [8] , [9] , [10] . In the optofluidic laser-based detection, ELISA is carried out in a microfluidic channel, which also forms an optical microcavity that provides the optical feedback for lasing. The laser onset time, that is, the time when laser emission starts to emerge, is employed as the sensing signal. In contrast to light intensity in the traditional ELISA, the laser onset time is inversely proportional to the enzyme concentration and hence the analyte concentration. In this article, we first elucidate the principle of the optofluidic laser-based ELISA, and then characterize the optofluidic laser performance. Finally, we present the dual-mode detection of interleukin-6 (IL-6) using commercial ELISA kits, where the sensing signals are simultaneously obtained by the traditional ELISA and the optofluidic laser-based ELISA. We observe that at relatively high IL-6 concentrations (≥100 fg ml −1 ), both sensing signals have the linear response to the IL-6 concentration in the log–log scale and follow each other closely. However, with further reduction in the analyte concentration, the traditional ELISA no longer responds. In contrast, the response from the optofluidic laser-based ELISA can extend to 1 fg ml −1 (38 aM), which represents a dynamic range of 6 orders of magnitude. Theoretical analysis of optofluidic laser-based ELISA The traditional sandwich format ELISA is illustrated in Fig. 1a . The fluorescent product from the enzyme–substrate reaction is determined by the Michaelis–Menten equation (1) (ref. 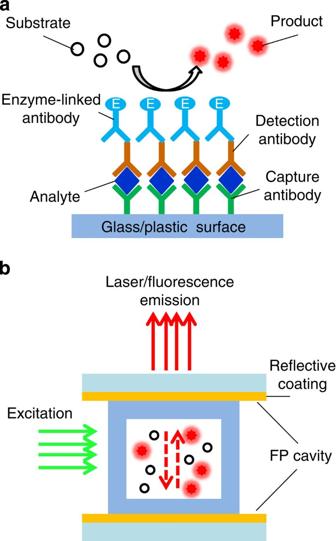Figure 1: Traditional ELISA and ELISA based on an optofluidic laser. (a) Details of traditional ELISA. (b) Optofluidic laser-based ELISA. The two mirrors form an FP optical cavity, within which a fluidic channel is inserted for sample delivery. The ELISA-related enzyme–substrate reaction occurs on the channel inner surface, which produces the fluorescent product that serves as the laser gain medium. Both regular fluorescence and laser emission can be collected through the top mirror of the FP cavity. 11 ): Figure 1: Traditional ELISA and ELISA based on an optofluidic laser. ( a ) Details of traditional ELISA. ( b ) Optofluidic laser-based ELISA. The two mirrors form an FP optical cavity, within which a fluidic channel is inserted for sample delivery. The ELISA-related enzyme–substrate reaction occurs on the channel inner surface, which produces the fluorescent product that serves as the laser gain medium. Both regular fluorescence and laser emission can be collected through the top mirror of the FP cavity. Full size image where [ P ] is the product concentration, k is a rate constant, [ E ] is the enzyme concentration in bulk solution (or the number of enzymes in a given volume in the case of ELISA) and t is the enzyme–substrate reaction time (or incubation time). For the traditional ELISA, the output fluorescence intensity is proportional to [ P ] (see Supplementary Note 1 for detailed analysis of the traditional ELISA). Figure 1b illustrates the concept of the optofluidic laser-based ELISA. The fluorescent products resulting from the enzyme–substrate reaction are used as the laser gain medium, whose concentration increases over time at a rate proportional to the number of the enzymes (and hence the analytes) attached to the microfluidic channel surface. Upon external excitation, the laser emission starts to emerge when the product reaches a threshold concentration. Instead of fluorescence intensity used in the traditional ELISA, the laser onset time is employed as the sensing signal, which is shown to be inversely proportional to the enzyme (and hence analyte) concentration. Therefore, the optofluidic laser ELISA is particularly useful to detect low concentrations of analytes. Furthermore, the traditional ELISA can be carried out simultaneously along with the optofluidic laser measurement. This dual-mode measurement significantly increases the ELISA performance. At high analyte concentrations, the results from the traditional ELISA will be used, whereas at low analyte concentrations where the traditional ELISA fails to detect, the results from the laser-based ELISA will be used. In the optofluidic laser-based ELISA (see Supplementary Note 1 for detailed analysis), there exists a lasing threshold ( I th ) determined by equation (2): where [ S ] 0 is the initial substrate concentration and γ is a fixed dimensionless parameter related to the characteristics of the optical cavity and the fluorescent product [12] , [13] . Note, all intensities described herein (such as I th ) are normalized to the saturation intensity, and therefore, dimensionless (see the discussion in Supplementary Note 1 ). When the external pump ( I pump ), which is fixed in the optofluidic laser-based ELISA, is below the lasing threshold, no laser emission is observed. With the increased [ P ] over time (equation (1)), I th continues to decrease. At the lasing onset time, τ , the product reaches the threshold concentration, [ P ] threshold , such that I pump = I th , the laser emission starts to emerge and increases according to equation (3): Supplementary Fig. 1 highlights the major spectral differences between fluorescence and laser emission. Supplementary Fig. 2 compares the traditional ELISA fluorescence and the laser emission arising from the same enzyme–substrate reaction. For fluorescence, no onset time exists. The fluorescence intensity increases over time with a unity slope in the log–log scale. In contrast, the laser emission has a clear-cut onset time, above which the lasing emission increases extremely rapidly (in the log–log scale). The laser onset time, τ , is determined by the following simple equation (4): where C is a constant for a given optofluidic laser. Thus, through an optofluidic laser, detection of the enzyme concentration [ E ] is converted to the laser onset time detection. It should be emphasized that the sensing signal, τ in equation (4), is inversely proportional to the enzyme concentration [ E ]. Therefore, the optofluidic laser method is particularly useful to detect low concentrations of analytes for which a small [ E ] and hence a large τ are anticipated. Owing to the extremely sharp slope in the laser output over time, the laser onset time can be determined accurately, which leads to a superior detection limit as shown later in the experimental part. Note that the above detection principle is applicable any types of optofluidic lasers, including the linear Fabry–Pérot (FP) cavity [14] , [15] , [16] , [17] , which we used in our study, the ring resonator [12] , [18] , [19] , [20] , [21] , [22] , and the distributed feedback laser cavity [23] , [24] , and so on. ELISA experimental setup We implemented the new ELISA detection scheme using an FP optofluidic laser. As illustrated in Fig. 1b (see also Supplementary Figs 3 and 4 ), a square glass capillary (1 × 1 mm for the inner channel and 150 μm for the wall thickness) was sandwiched between two gold mirrors (reflectivity=0.70 and 0.8 for the top and bottom mirror, respectively) that formed an FP laser cavity. The samples and reagents were flowed through the capillary and the enzyme–substrate reaction could take place in either bulk solution, or, in the case of ELISA, on the capillary inner wall. The fluorescent product filled the entire capillary cross section and served as the laser gain medium. The optofluidic laser was excited with a pulsed optical parametric oscillator (OPO, 5 ns pulse width, 20 Hz repetition rate) at 532 nm. Both fluorescence and laser emission were collected simultaneously through the top mirror and sent to a spectrometer for analysis. Details of the experimental setup can be found in Methods. Characterization of the optofluidic laser We first characterized the optofluidic laser through the enzyme–substrate reaction taking place in bulk solution, which allows for easy and accurate control of the enzyme concentration in reaction, thus providing quantitative information for us to verify the theoretical analysis and understand how the optofluidic laser responds to the enzyme–substrate reaction. It is a critical step towards the final optofluidic laser-based ELISA, in which the enzyme-substrate reaction occurs on the solid inner surface of the capillary. In our experiment, we prepared the fluorescent product by mixing a relatively high concentration of horseradish peroxidase (HRP, Thermo Scientific, a commonly used enzyme in ELISA) with QuantaRed (Thermo Scientific, a commonly used substrate in ELISA) in a vial (see Methods for details of materials and experimental procedures). After short reaction time, the solution was flowed through the laser cavity and excited by the OPO. Strong lasing emission peaks emerged and were superimposed on the red-side of the product fluorescence spectrum ( Fig. 2 ). The threshold was ~320 μJ mm −2 , well within the capability of an OPO. To the best of our knowledge, this is the first demonstration of an optofluidic laser mediated by enzyme–substrate reaction. For comparison, the emission of QuantaRed alone without HRP is also plotted in Fig. 2 , showing much weaker and featureless spectrum. Figure 3 presents the lasing emission of the product with various enzyme–substrate reaction times. 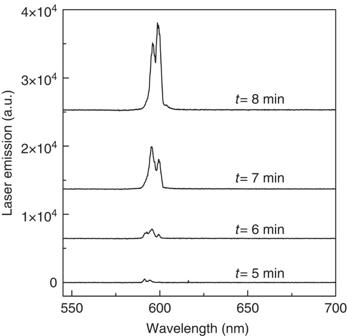Figure 3: Lasing spectra versus HRP-QuantaRed reaction time. Laser emission increases with increased enzyme–substrate reaction time. The HRP concentration was 4 ng ml−1. The pump energy density was fixed at 1,244 μJ mm−2per pulse. The broad fluorescence spectra are subtracted. The curves are vertically shifted for clarity. 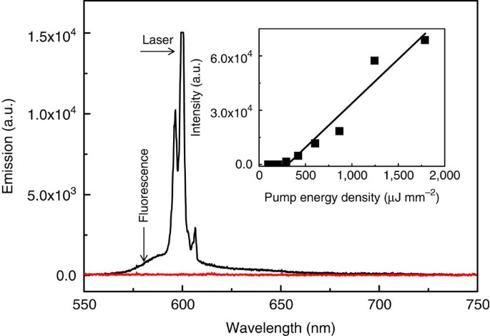With the increased reaction time, the product concentration increases and hence the laser output, as predicted by equation (3). Figure 2: Laser emission from the product of enzyme–substrate reaction. Black curve, strong laser emission peaks are superimposed on the broad spectrum of fluorescence, both of which resulted from the product after 30 min of the HRP-QuantaRed reaction with the HRP concentration of 4 ng ml−1. The samples were flowed through the FP cavity and were excited by an OPO at 532 nm with a pump energy density of 1,244 μJ mm−2. Inset, spectrally integrated laser output (after removal of fluorescence) between 575 nm and 625 nm as a function of pump energy density. The solid line is the linear fit above the lasing threshold of 320 μJ mm−2. Red curve, for comparison, no laser emission could be generated from QuantaRed alone in the absence of HRP under otherwise the same conditions as the black curve. Figure 2: Laser emission from the product of enzyme–substrate reaction. Black curve, strong laser emission peaks are superimposed on the broad spectrum of fluorescence, both of which resulted from the product after 30 min of the HRP-QuantaRed reaction with the HRP concentration of 4 ng ml −1 . The samples were flowed through the FP cavity and were excited by an OPO at 532 nm with a pump energy density of 1,244 μJ mm −2 . Inset, spectrally integrated laser output (after removal of fluorescence) between 575 nm and 625 nm as a function of pump energy density. The solid line is the linear fit above the lasing threshold of 320 μJ mm −2 . Red curve, for comparison, no laser emission could be generated from QuantaRed alone in the absence of HRP under otherwise the same conditions as the black curve. Full size image Figure 3: Lasing spectra versus HRP-QuantaRed reaction time. Laser emission increases with increased enzyme–substrate reaction time. The HRP concentration was 4 ng ml −1 . The pump energy density was fixed at 1,244 μJ mm −2 per pulse. The broad fluorescence spectra are subtracted. The curves are vertically shifted for clarity. Full size image In Fig. 4 , we systematically investigated the laser output characteristics for various HRP concentrations. Again each enzyme–substrate mixture was prepared in a vial and the flowed through the optofluidic laser cavity (see Methods for details of materials and experimental procedures). 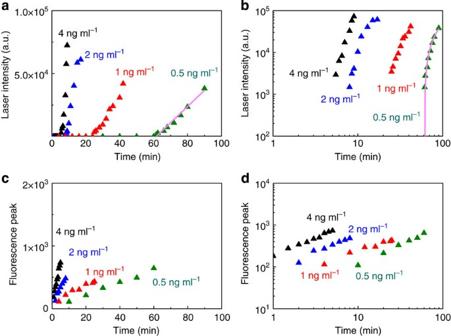Figure 4: Laser intensity and fluorescence peak as a function of reaction time. (a,b) Spectrally integrated laser output as a function of reaction time in the linear–linear and log–log scale. Spectral integration takes place between 575 nm and 625 nm. The solid lines in (a) and (b) are the linear fit above the lasing threshold for one of the measurements plotted in the linear–linear and log–log scale, respectively. The initial slope near the laser onset time in the log–log scale is 70. The lasing onset times extracted through the curve fit are plotted inSupplementary Fig. 5. The pump energy density was fixed at 1,244 μJ mm−2per pulse. (c,d) Fluorescence peak around 587 nm before the lasing was achieved as a function of reaction time in the linear–linear and log–log scale. Both laser spectra and fluorescence spectra were obtained under the same condition (except at different enzyme-substrate reaction times). The HRP concentration was 4 ng ml−1, 2 ng ml−1, 1 ng ml−1and 0.5 ng ml−1, respectively. Figure 4a shows the spectrally integrated laser intensity as a function of reaction time in the linear–linear scale for the HRP concentration ranging from 0.5 to 4 ng ml −1 . For a high HRP concentration (for example, 4 ng ml −1 ), the laser emission increases rapidly. For a low HRP concentration (for example, 0.5 ng ml −1 ), the laser emission increases at a much slower pace due to the slower reaction rate. The laser onset characteristics may be better revealed in the log–log scale in Fig. 4b . First, there is clearly an onset time for each HRP concentration, below which no emission is detected. Second, the laser output increases drastically with a steep slope near the laser onset time, which results from the discontinuity caused by the threshold nature in the laser output curve. For example, the solid line in Fig. 4b shows that near the laser onset time the slope is ~70, meaning that within only 2 min (that is, 3.3% of the laser onset time of 62 min), the lasing signal increases by a factor of 10. The sharp increase of the laser emission is critical to accurately determining the onset time. All these results agree qualitatively well with Supplementary Fig. 2c and d predicted by equation (2). In contrast, Fig. 4c,d shows the fluorescence obtained before the corresponding lasing emission was achieved. As expected, the fluorescence emission emerges immediately when enzyme–substrate reaction starts and no emission onset time is observed. When plotted in the log–log scale, all curves are parallel to each other with a unity slope, as expected from equation (1) (see Supplementary Fig. 2a,b ). Note that after the lasing emission was achieved, residual fluorescence could still be observed (see, for example, Fig. 2 ). However, since the laser emission significantly affects the dynamics of fluorescence, the fluorescence accompanying the laser emission cannot be used in our fluorescence analysis. As such, Fig. 4c,d only plots the fluorescence data before the corresponding laser emission was achieved. Figure 4: Laser intensity and fluorescence peak as a function of reaction time. ( a , b ) Spectrally integrated laser output as a function of reaction time in the linear–linear and log–log scale. Spectral integration takes place between 575 nm and 625 nm. The solid lines in ( a ) and ( b ) are the linear fit above the lasing threshold for one of the measurements plotted in the linear–linear and log–log scale, respectively. The initial slope near the laser onset time in the log–log scale is 70. The lasing onset times extracted through the curve fit are plotted in Supplementary Fig. 5 . The pump energy density was fixed at 1,244 μJ mm −2 per pulse. ( c , d ) Fluorescence peak around 587 nm before the lasing was achieved as a function of reaction time in the linear–linear and log–log scale. Both laser spectra and fluorescence spectra were obtained under the same condition (except at different enzyme-substrate reaction times). The HRP concentration was 4 ng ml −1 , 2 ng ml −1 , 1 ng ml −1 and 0.5 ng ml −1 , respectively. Full size image Comparison between Fig. 4a–d suggests that the time-dependent laser emission reflects the underlying enzyme–substrate reaction. This can further be verified in Supplementary Fig. 5 when we plot the inverse of the laser onset time and of the time for the fluorescence peak to reach a certain value (for example, 200 counts) for various HRP concentrations. Both curves follow closely each other. Linear dependence in the log–log scale shows the same slope of 1.2, in good agreement with the unity slope predicted in equations (1) and (4). Therefore, the laser onset time can indeed be used as the sensing signal to quantify the enzyme concentration (or the number of enzymes in a given volume). Optofluidic laser for dual-mode ELISA detection Our final goal is to develop the optofluidic laser for dual-mode ELISA detection, where the enzyme–substrate reaction occurs on the inner surface of the microfluidic channel. For these experiments, we used a biomarker, Human Interleukin 6 (Human IL-6), as a model system. We purchased commercial Human IL-6 DuoSet ELISA Kit (R&D Systems, no. DY206), which consisted of capture antibody, analytes (Human IL-6, ~26 kDa), detection antibody and streptavidin-labelled HRP. Blocking buffer and substrate (QuantaRed) were purchased from Thermo Scientific. We followed exactly the instructions and ELISA protocols provided by the vendor, except the last readout step, where both the laser emission and the fluorescence from HRP-QuantaRed reaction products were detected. See Methods for details of materials and experimental procedures. Supplementary Fig. 6 shows two emission spectra from ELISA occurring inside the optofluidic laser cavity when the laser just reaches its threshold. Small sharp laser peaks start to emerge above the broad fluorescence spectra. Although the spectra are virtually identical, they were actually obtained at different enzyme–substrate reaction times due to different laser onset times caused by different IL-6 concentrations. 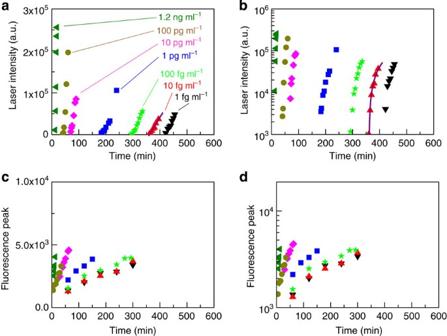Figure 5: Dual-mode ELISA measurement of Human IL-6 with the optofluidic laser. (a,b) Spectrally integrated laser output from 575 nm to 625 nm as a function of reaction time for various concentrations of IL-6 in the linear–linear and linear–log scale. The solid lines in (a) and (b) are the linear fit above the lasing threshold for one of the measurements plotted in the linear–linear and linear–log scale, respectively. (c,d) Fluorescence peak around 587 nm before the lasing was achieved as a function of reaction time for various concentrations of IL-6 in the linear–linear and linear–log scale. Both laser spectra and fluoresce spectra were obtained under the same condition (except at different enzyme-substrate reaction times). The detailed fluorescence spectra for 1 fg ml−1and 10 fg ml−1are presented inSupplementary Fig. 7. The pump energy density was fixed at 1,870 μJ mm−2per pulse. Figure 5a,b shows the spectrally integrated intensity of the ELISA laser emission as a function of enzyme–substrate reaction time. Distinct difference in the laser onset time can be seen among different IL-6 concentrations, even at the level of 1 fg ml −1 . In sharp contrast, the fluorescence obtained under the same condition shows diminished difference with the decreased analyte concentration ( Fig. 5c,d ). When the IL-6 concentration was below 100 fg ml −1 , the fluorescence started to level off and became indistinguishable (see Supplementary Fig. 7 ). Note, as discussed previously in Fig. 4c,d , only the fluorescence before the corresponding laser emission was achieved is displayed in Fig. 5c,d , and used in fluorescence data analysis. Figure 5: Dual-mode ELISA measurement of Human IL-6 with the optofluidic laser. ( a , b ) Spectrally integrated laser output from 575 nm to 625 nm as a function of reaction time for various concentrations of IL-6 in the linear–linear and linear–log scale. The solid lines in ( a ) and ( b ) are the linear fit above the lasing threshold for one of the measurements plotted in the linear–linear and linear–log scale, respectively. ( c , d ) Fluorescence peak around 587 nm before the lasing was achieved as a function of reaction time for various concentrations of IL-6 in the linear–linear and linear–log scale. Both laser spectra and fluoresce spectra were obtained under the same condition (except at different enzyme-substrate reaction times). The detailed fluorescence spectra for 1 fg ml −1 and 10 fg ml −1 are presented in Supplementary Fig. 7 . The pump energy density was fixed at 1,870 μJ mm −2 per pulse. 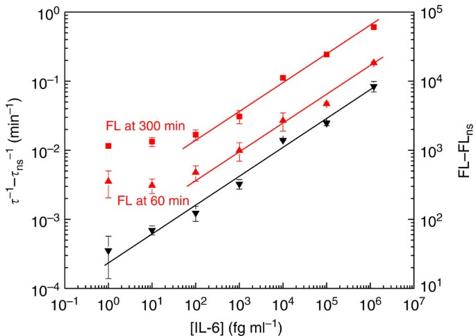Figure 6:Dual-mode sensing signal versus IL-6 concentration. Sensing signals, laser onset time for the optofluidic laser-based ELISA (black curve, leftYaxis) and fluorescence peak for the traditional ELISA (red curves, rightYaxis), as a function of IL-6 concentration extracted fromFig. 5. The laser onset time is defined as the time when the laser intensity reaches 1,000 (counts from CCD) inFig. 5. The fluorescence signals at 60 min and 300 min are defined as the peak values obtained at 60 min and 300 min of reaction time, respectively. The solid lines are the linear fit in the log–log scale for the IL-6 concentrations above 1 fg ml−1(for optofluidic laser-based ELISA) and above 100 fg ml−1(for traditional ELISA). Owing to saturation of the fluorescence at high IL-6 concentrations, the fluorescence peak values for 100 pg ml−1and 1.2 ng ml−1at 60 min are obtained by linearly extrapolating the corresponding curves inFig. 5cto 60 min. Similarly, the fluorescence peak values for 1 pg ml−1, 10 pg ml−1, 100 pg ml−1and 1.2 ng ml−1at 300 min are obtained by linearly extrapolating the corresponding curves inFig. 5cto 300 min. Error bars are obtained based on triplicate measurements. FL, fluorescence. Full size image Figure 6 plots the sensing signal from the optofluidic laser-based ELISA (that is, the laser onset time) and the traditional ELISA (that is, the fluorescence peak value at 60 min of reaction time) after removal of non-specific binding (that is, [ IL-6 ]=0 fg ml −1 ) background (see Supplementary Fig. 8 ). The reason to choose the fluorescence at 60 min is because for most of the IL-6 concentrations under study, the laser emission has not occurred yet, and therefore, fluorescence can be measured directly without linear extrapolation. Figure 6 clearly shows that at relatively high analyte concentrations (≥100 fg ml −1 ), both types of sensing signals follow each other closely and decrease with nearly the same linear slope (in the log–log scale) when the IL-6 concentration is lowered. In this regime, both the traditional and the optofluidic laser-based ELISA can be used to quantify analytes. However, with further reduction in the IL-6 concentration (~10 fg ml −1 ), the fluorescence signal from the traditional ELISA starts to deviate significantly from the linear response (in the log–log scale). Similar behaviour can also be seen with even longer reaction time (300 min, see Fig. 6 ). In contrast, the response of the optofluidic laser-based ELISA can extend to 1 fg ml −1 (38 aM), which significantly increases the dynamic range to 6 orders of magnitude (1 fg ml −1 –1.2 ng ml −1 ). For comparison, the dynamic range of various commercial ELISA kits/protocols is presented in Supplementary Fig. 9 . Figure 6: Dual-mode sensing signal versus IL-6 concentration . Sensing signals, laser onset time for the optofluidic laser-based ELISA (black curve, left Y axis) and fluorescence peak for the traditional ELISA (red curves, right Y axis), as a function of IL-6 concentration extracted from Fig. 5 . The laser onset time is defined as the time when the laser intensity reaches 1,000 (counts from CCD) in Fig. 5 . The fluorescence signals at 60 min and 300 min are defined as the peak values obtained at 60 min and 300 min of reaction time, respectively. The solid lines are the linear fit in the log–log scale for the IL-6 concentrations above 1 fg ml −1 (for optofluidic laser-based ELISA) and above 100 fg ml −1 (for traditional ELISA). Owing to saturation of the fluorescence at high IL-6 concentrations, the fluorescence peak values for 100 pg ml −1 and 1.2 ng ml −1 at 60 min are obtained by linearly extrapolating the corresponding curves in Fig. 5c to 60 min. Similarly, the fluorescence peak values for 1 pg ml −1 , 10 pg ml −1 , 100 pg ml −1 and 1.2 ng ml −1 at 300 min are obtained by linearly extrapolating the corresponding curves in Fig. 5c to 300 min. Error bars are obtained based on triplicate measurements. FL, fluorescence. Full size image One question may arise as to whether the traditional ELISA can achieve the same dynamic range and detection limit as the laser-based ELISA, given sufficient reaction time. Unfortunately, the presence of the laser emission in our current setup precludes accurate measurement of the fluorescence peak value beyond the lasing onset time. To completely eliminate the interference from the laser emission, in a control experiment presented in Supplementary Fig. 10 both mirrors in Fig. 1b were removed from the microfluidic channel so that the traditional ELISA could be carried out (see details in Methods). For short reaction time (20 min), the fluorescence sensing signal resembles closely that in Fig. 6 . For the fluorescence taken at 480 min (close to the laser onset time for 0 fg ml −1 ), the sensing dynamic range is severely impaired by the saturation of the enzyme–substrate reaction (that is, nearly all substrates were converted to the products). Furthermore, the fluorescence-sensing signal deviates substantially from the normal response to the change in the analyte concentration, rendering the response curve virtually useless in practice. Our work has demonstrated the unique capability of the optofluidic laser in sensitively detecting analytes with a significantly improved detection limit and dynamic range over the traditional ELISA. The optofluidic laser-based ELISA works particularly well when the analyte concentration (and hence enzyme concentration [ E ]) is low. This is due to the fact that the laser onset time τ is inversely proportional to [ E ] (equation (4)). The results presented in this article suggest that the dual-mode measurement can be implemented. At high analyte concentrations, the results from the traditional ELISA (which can be obtained with short enzyme–substrate reaction time) will be used, whereas at low analyte concentrations where the traditional ELISA fails to detect, the results from the laser-based ELISA will be used. Since the sensing signals from both the traditional ELISA and the optofluidic laser-based ELISA follow each other closely (see Fig. 6 ), they can easily be converted and stitched together seamlessly. Such combination will enable an excellent detection limit with a large dynamic range. Moreover, in contrast to the fluorescence intensity-based detection, whose signal is proportional to the total number of fluorescent products in a detection volume, the laser onset time depends on the product concentration. Therefore, the optofluidic laser becomes attractive with microfluidic systems, where the total number of analytes, enzymes and fluorescent molecules decreases significantly compared with conventional fluidic systems. Furthermore, our analysis shows that the surface density of the non-specifically bound enzymes in the current optofluidic laser is ~1.6 × 10 7 cm −2 , ~40 times higher than required for digital ELISA [3] , [7] (see Supplementary Note 2 for detailed calculation), suggesting that the optofluidic laser-based ELISA may work better in an environment with relatively high non-specific bindings, which is important when we test actual analytes in body fluids such as blood and saliva. Finally, the principle of the optofluidic laser-based ELISA can readily be extended to any other types of laser cavities such as ring resonators (see Supplementary Note 3 , and Supplementary Figs 11 and 12 for optofluidic ring resonator laser-based ELISA detection). Such versatility is highly desirable to optimize the optofluidic laser for best detection performance and to accommodate different biological and biochemical needs. However, it should be noted that in the current configuration, the laser onset time is long. Especially for the detection of low analyte concentrations, reaction time over 100 min is needed. Such a drawback can potentially be overcome by increasing the surface-to-volume ratio with micro/nanostructures (like microposts) within the laser cavity or by using cavities with higher Q-factors. Furthermore, although 1 fg ml −1 of analyte has been detected in the current work, there is still plenty of room for improvement in the detection limit in the optofluidic laser-based ELISA. The fundamental limit will mainly be determined by the level and variations of the non-specific bindings and the accuracy in laser onset time measurement. In the near future, shortening the overall assay time, pushing the detection limit and carrying out detection of analytes in serological samples will be pursued. Device fabrication The top and bottom mirrors were fabricated by respectively coating a 40 nm and 150 nm thick layer of gold to 500 μm thick glass wafers (Solitaire). The reflectivity was ~0.7 and 0.8 for the top and bottom mirror, respectively. The mirrors were then glued onto the top and bottom an array of square-shaped glass capillaries (Friedrich & Dimmock Inc., 1 mm × 1 mm inner cross section, 150 μm wall thickness) using UV-curable adhesives to form FP optofluidic laser cavities. See Supplementary Fig. 3 for illustrations. Experimental setup The experimental setup is shown in Supplementary Fig. 4 . The optofluidic laser filled with the solution was pumped by a pulsed OPO from Continuum at 532 nm with a 5-ns pulse width and a 20-Hz repetition rate. The lasing emission and fluorescence were collected by a multimode fibre and subsequently transmitted to a spectrometer (Ocean Optics, HR4000). The spectra were acquired using the built-in software coming with Ocean Optics. The acquisition time was 0.5 s for bulk solution measurements in Figs 2 , 3 , 4 and 2 s for ELISA measurements in Figs 5 and 6 . During the experiment, the solution was withdrawn into the capillary with a syringe pump (Harvard Apparatus 55–4140). Samples and reagents For bulk solution measurement presented in Figs 2 , 3 , 4 in the main text, HRP and substrates were purchased from Thermo Scientific. A stock of 1 mg ml −1 HRP solution was prepared by dissolving salt-free lyophilized HRP powder (product no. 31490) in 0.1 M potassium phosphate buffer (pH 6.0) at room temperature. Then, HRP solutions with concentrations of 0.4 μg ml −1 , 0.2 μg ml −1 , 0.1 μg ml −1 and 50 ng ml −1 were prepared by diluting the stock solution with the same buffer. The substrate kit (product no. 15159) contained QuantaRed10-acetyl-3,7-dihydroxyphenoxazine (ADHP) Concentrate, QuantaRed Enhancer Solution and QuantaRed Stable Peroxide Solution. The working substrate solution was prepared by mixing 2 μl QuantaRed concentrate, 100 μl Enhancer Solution and 100 μl Stable Peroxide Solution at room temperature. The final mixture of HRP and substrate was prepared by mixing HRP solution with substrate solution at a volume ratio of 1:99. For ELISA measurement in Figs 5 and 6 , Human IL-6 DuoSet ELISA Kit (DY206), ELISA Plate-coating buffer (DY006), wash buffer (WA126) and reagent diluent (DY995) were purchased from R&D Systems. Blocking buffer BSA in PBS (product no. 37525) and QuantaRed Enhanced Chemifluorescent HRP Substrate (product no. 15159) were purchased from Thermo Scientific. The reagents were prepared according to the procedure described in the kits’ user manuals. First, the stock wash buffer and reagent diluent were diluted with Milli-Q water to achieve 1 × working solutions. Then, the capture antibody working solution of 12 μg ml −1 was prepared by diluting with PBS buffer. The detection antibody working solution of 0.4 μg ml −1 was prepared by diluting with the reagent diluent. The Human IL-6 standard was diluted to a desired concentration by adding the reagent diluent. The HRP-labelled streptavidin (SAv-HRP) working solutions was prepared by diluting 10 μl of the SAv-HRP stock solution from DY206 kit with 190 μl of the reagent diluent. The working substrate solution of QuantaRed was prepared as described in the previous paragraph. The stock blocking buffer solution (10% BSA in PBS) was further diluted with PBS to achieve 1% BSA working blocking buffer solution. Procedures for the optofluidic laser characterization First, 198 μl of substrate solution was mixed with 2 μl of HRP solution in a vial. Then, the square capillary was filled with the mixture, which was optically pumped with the OPO. The emission spectrum was recorded over time. Upon completion of the measurement, the capillary was rinsed with potassium phosphate buffer, followed by another rinse with the wash buffer solution. After this regeneration step, the capillary was ready for another measurement. Procedures for optofluidic laser-based ELISA measurement The overall procedures were adapted from those listed in the user manual accompanying the Human IL-6 DuoSet ELISA Kit from R&D Systems. They consisted of seven steps. Step 1: the square capillary was filled with the capture antibody solution and incubated for 10 min. Then it was filled with the wash buffer and incubated for 10 min. Finally, the capillary was filled with the blocking buffer (1% BSA in PBS) and incubated for 10 min. Step 2: the solution containing the analyte (IL-6) was flowed through the capillary and incubated for 20 min, followed by the wash buffer and additional 10 min of incubation. Step 3: the detection antibody solution was flowed through the capillary and incubated for 10 min, followed by the wash buffer and additional 10 min of incubation. Step 4: the SAv-HRP solution was flowed through the capillary and incubated for 10 min, followed by the wash buffer and additional 20 min of incubation. Step 5: the capillary was filled with the substrate solution of QuantaRed. The OPO was turned on to excite the solution and the emission spectrum was recorded over time. Step 6: upon completion of the measurement, the capillary was filled with the wash buffer and incubated for 20 min. Step 7: the capillary inner surface was etched slightly by 0.1% hydrofluoric acid for 2 min, which removed the residual molecules attached to the capillary surface. Then the capillary was filled with the wash buffer and incubated for 5 min. Finally, the capillary was filled the ELISA Plate-coating Buffer PBS (R&D Systems cat. no. DY006) for overnight. After this regeneration step, the capillary was ready for the next round of measurement. All measurements reported in this article were performed at room temperature and the solution was withdrawn into the capillary at a flow rate of 100 μl min −1 with a syringe pump. Step 7 was always performed before Step 1 of the first cycle of experiment using a square capillary. Procedures for traditional ELISA measurement with a CW laser Experimental procedures, reagent concentrations, ELISA protocols and capillaries in the ELISA fluorescence measurement were the same as for the optofluidic laser-based ELISA experiment described in Methods. However, both mirrors in the FP cavity were removed to avoid lasing. A CW laser at 532 nm (JDS Uniphase), which has better power stability than the OPO, was used to excite the product with a laser diameter of ~1 mm and power of 90 μW. The fluorescence was collected from the same excitation spot and recorded with a spectrometer (Ocean Optics, HR4000) using 2 s of acquisition time. The results are presented in Supplementary Fig. 10 . How to cite this article: Wu, X. et al. Optofluidic laser for dual-mode sensitive biomolecular detection with a large dynamic range. Nat. Commun. 5:3779 doi: 10.1038/ncomms4779 (2014).